Receptor mimicry by antibody F045–092 facilitates universal binding to the H3 subtype of influenza virus Influenza viruses present a significant health challenge each year, as in the H3N2 epidemic of 2012–2013. Here we describe an antibody, F045–092, that possesses broadly neutralizing activity against the entire H3 subtype and accommodates the natural variation and additional glycosylation in all strains tested from 1963 to 2011. Crystal structures of F045–092 in complex with HAs from 1975 and 2011 H3N2 viruses reveal the structural basis for its neutralization breadth through insertion of its 23-residue HCDR3 into the receptor-binding site that involves striking receptor mimicry. F045–092 extends its recognition to divergent subtypes, including H1, H2 and H13, using the enhanced avidity of its IgG to overcome lower-affinity Fab binding, as observed with other antibodies that target the receptor-binding site. This unprecedented level of antibody cross-reactivity against the H3 subtype can potentially inform on development of a pan-H3 vaccine or small-molecule therapeutics. Influenza virus infects millions annually and causes severe illness and economic distress. The constant threat of a novel pandemic influenza virus looms large as with the emergence in 2009 of the H1N1 swine flu that antigenically closely resembled the 1918 H1N1 Spanish flu, which resulted in death of ~50 million people worldwide. Fortunately, the novel 2009 H1N1 virus was much less severe and subsequently became the circulating seasonal H1 strain. The H3N2 virus in 2012–2013 was more virulent than usual and caused epidemics in the northeastern United States [1] . The unpredictable epidemic and pandemic potential of these viruses underscores the need for broad-spectrum therapy. To combat flu infections, small molecules are available that target the neuraminidase surface glycoprotein on influenza virus, but the effectiveness of these drugs is diminishing [2] , [3] and underscores the need for new classes of drugs. Vaccine therapy remains the best means as a preventative countermeasure from flu infections. However, vaccine strains must be reformulated almost every year to stay ahead of the ever-changing virus and may not provide protection if they are an inadequate match to the dominant circulating virus. Much of the challenge in raising a broadly neutralizing antibody response against influenza by a universal flu vaccine arises from the diversity and hypervariability of the haemagglutinin (HA) surface glycoprotein. There are currently 18 identified HA subtypes (H1–H18) of influenza A viruses, where aquatic birds act as the primary reservoir. Among these, only the H1 and H3 subtypes currently circulate in humans although sporadic cases of H5, H7, including the most recent H7N9 outbreak [4] , [5] , and H9 have caused deaths and severe illness. Thus, emerging viruses are carefully monitored for any propensity to acquire human-to-human transmission that would increase the potential to cause a human pandemic. Despite extensive sequence diversity across HA subtypes, viral attachment to terminal sialic acid glycans on host cells is a conserved function of the HA that initiates viral infection [6] , [7] , although the newly discovered bat H17 and H18 HAs appear to be exceptions [8] , [9] , [10] . The HA interaction with sialosides is very weak ( K d ~mM) and the virus is thus reliant on multivalency to achieve high enough affinity for productive receptor binding and subsequent receptor-mediated endocytosis. HA is synthesized as a single polypeptide precursor (HA0) that assembles into trimers, which mature after proteolytic cleavage by host proteases between the HA1 and HA2 subunits to produce a pH-dependent metastable intermediate. In structural and functional terms, HA can be divided into a membrane-proximal ‘stem’, which constitutes the core fusion machinery that is triggered by low pH in the endosomes [11] , and a membrane-distal ‘head’, which contains the receptor-binding site (three per HA trimer). The receptor-binding site is a broad and shallow pocket located at the apex of the HA head and its outer ridges are formed primarily by four loops named after their locations in the HA sequence: the 130 loop, 150 loop, 190 helix and 220 loop. Blocking HA–receptor interactions can prevent infection by influenza virus. However, despite the functional conservation of receptor binding, the design of entry inhibitors to the HA still remains a significant challenge due to the shallowness of the receptor-binding pocket and sequence divergence within and across HA subtypes. Nevertheless, a number of HA receptor-binding-site-targeted antibodies have been structurally characterized that have broader-spectrum activity against a single subtype [12] , [13] , [14] , [15] or across multiple subtypes [16] , [17] , thus suggesting that the receptor-binding pocket is indeed a site of vulnerability on HA [18] . The breadth of recognition of these antibodies is surprising as it was popularly believed until recently that the HA head could only elicit strain-specific antibodies. All of these antibodies that target the receptor-binding site insert a single complementarity determining region (CDR) loop (HCDR2 or HCDR3) into the receptor-binding site to prevent viral-host recognition; however, due to the larger footprints of antibodies in comparison to the sialic acid receptor, they invariably contact variable residues on the outer edges of the receptor-binding pocket and, hence, have limited breadth compared to stem-directed antibodies. Here, we describe crystal structures of antibody F045–092 bound to divergent HAs from the 1975 and 2011 H3 subtype. The antibody was selected from a phage-displayed library, derived from human B lymphocytes, and was reported to have activity against a panel of H3 strains from 1968 to 2004 and possesses neutralizing activity against all H3N2 viruses that were tested within this time span as well as certain H1N1, H2N2 and H5N1 viruses [19] . The antibody contacts a minimal epitope in the HA receptor-binding site primarily by insertion of its 23-residue HCDR3 and achieves exceptional receptor mimicry. Full coverage of an entire subtype by interaction with the receptor-binding site is of great significance and the structural information from the complexes may potentially advance the design of novel small-molecule inhibitors as well as inform on the formulation of immunogens as vaccine candidates against H3 viruses. 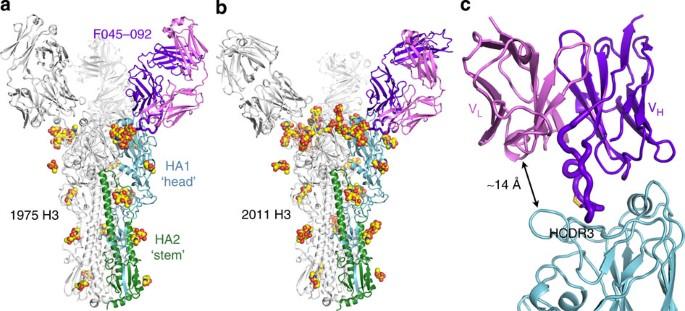Figure 1: Antibody F045–092 binds the influenza HA receptor-binding site. Crystal structures of F045–092 Fab in complex with (a) Vic1975/H3 HA and (b) Vic2011/H3 HA. One Fab-HA protomer is coloured with HA1 in light blue, HA2 in green, the Fab heavy chain in purple and the Fab light chain in pink. Glycans are shown as spheres with carbon in yellow, oxygen in red and nitrogen in blue. (c) F045–092 binds HA using only its heavy chain and inserts its HCDR3 into the HA receptor-binding site. The HCDR3 contains a disulphide bridge, which is shown in yellow sticks. Binding affinity of F045–092 against HAs To further profile its breadth, binding of F045–092 Fab and IgG was measured against a panel of HAs that encompass representative strains from nearly all HA subtypes by bio-layer interferometry ( Table 1 and Supplementary Table 1 ). F045–092 has heterosubtypic activity and binds HAs from the H1, H2, H3 and H13 subtypes. Most notably, F045–092 Fab binds all 13 representative HAs from strains from the H3 subtype that span five decades from 1963 to 2011, including the 2012–2013 H3 vaccine strain A/Victoria/361/2011 (Vic2011/H3). Although the HAs of some strains are strongly bound by the Fab ( K d ~5–50 nM), others have only moderate to weak binding ( K d ~50 nM to 5 μM), some of which are outside the threshold thought to be necessary for effective neutralization ( K d <250 nM) [17] . However, the bivalent F045–092 IgG shows increased affinity through avidity ( K d <20 nM) that significantly improves F045–092 binding to all strains compared with the monovalent Fab ( Table 1 ). These IgG-binding data are consistent with the reported neutralization data [19] . Avidity has also been observed, and now appears to be a common feature, for other receptor-binding-site-targeted antibodies [16] , [17] as the close packing and high density of HA trimers on viruses [20] likely promotes and facilitates bivalent binding by IgG. Moreover, binding of F045–092 was tested against strains beyond the years that were tested for neutralization (1968–2004) [19] . Despite further antigenic variation, the more recent strains (2007–2011) are bound with high affinity by IgG, indicating that F045–092 may truly be a pan-H3 antibody. Table 1 Binding breadth of F045–092 Fab and IgG to influenza HA subtypes and strains. 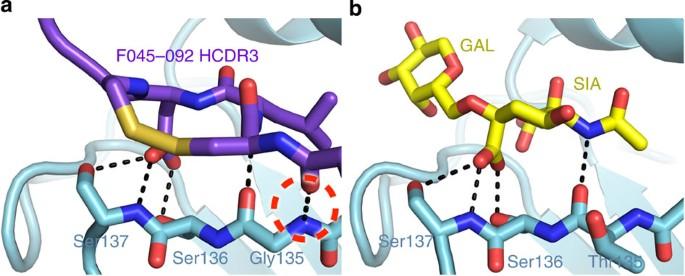Figure 2: Receptor-binding site recognition by F045–092 to Vic1975/H3 in comparison to the α2,6 sialoglycan receptor. (a) F045–092 inserts its HCDR3 into the HA receptor-binding site. The carboxylate side chain of F045–092 Asp100e overlaps with the (b) carboxylate moiety of the sialic acid of the α2,6 sialoglycan receptor (PDB 2YP4) and uses identical hydrogen-bonding interactions, which are shown as black dashed lines. An additional hydrogen bond between the main chains of F045–092 and HA is circled in red dashed lines. The Leu100d side chain of F045–092 overlaps with the acetamide moiety of sialic acid. Full size table Crystal structures of the F045–092–HA complexes To decipher the structural basis for this pan-H3 recognition by F045–092, crystal structures of the F045–092 Fab in complex with the HAs from the A/Victoria/3/1975 (Vic1975/H3) and A/Victoria/361/2011 (Vic2011/H3) viruses were determined at 2.75 Å and 6.50 Å resolution ( Table 2 ). In addition, crystal structures of the F045–092 Fab and the unliganded Vic2011/H3 HA were determined at 1.50 Å and 1.75 Å resolution ( Table 2 ), respectively, and served as high-resolution starting models for refinement of the Fab–HA complexes. In the crystal asymmetric unit, one copy of the Fab is bound to one HA protomer of the HA trimer in the F045–092–Vic1975/H3 complex. The HA protomer and the Fab variable domain are well ordered, as judged from the electron density, whereas the Fab constant domain appears to be disordered, as frequently found in other Fab–HA complexes [14] , [17] , [21] , [22] , [23] due to flexibility of the elbow region connecting the Fab variable and constant domains [24] . The asymmetric unit of the F045–092–Vic2011/H3 complex contains two HA trimers bound by six copies of the Fab. Despite the moderate resolution, the HA and Fab molecules can be clearly observed in the electron density maps ( Supplementary Fig. 1 ). All six Fab variable domains similarly recognize HA, but have a slight difference in approach angle on average (~14° rotation) in comparison to the F045–092–Vic1975/H3 complex; at this stage, these values are still qualitative given that we are comparing different resolution structures. No major conformational changes were observed between the apo and bound Fab in either complex. There is also good structural agreement between the HAs from the Vic1975/H3 and Vic2011/H3 complexes (Cα root mean squared deviation (r.m.s.d.) of ~0.4 Å) despite their divergence over 36 years, which amounted to 62 amino-acid mutations in the HA ectodomain. Table 2 Data collection and refinement statistics. Full size table The F045–092 Fab binds near the apex of HA to a single protomer of the HA trimer ( Fig. 1 ) and contacts portions of antigenic sites A, B and D [25] . The interactions are mediated only through the heavy chain using all three of its CDR loops, whereas the light chain is positioned ~14 Å away from the HA main chain and only comes within ~10 Å of a conserved glycan at Asn165 from a neighbouring HA protomer in the trimer ( Fig. 1c ). Indeed, the heavy chain CDRs form a ridge and protrude much further from the Fab core than the CDRs from the light chain ( Supplementary Fig. 2 ). F045–092 reaches into the receptor-binding site through insertion of its long 23-residue HCDR3, which notably contains an intrachain disulphide separated by only two amino acids ( Fig. 2a ). This unusual disulphide in HCDR3 has only been seen in only a few other antibody structures [26] , [27] , [28] . As the HCDR3 and sialoglycan receptor bind to the same specificity pockets in the receptor-binding site ( Fig. 2b ), the F045–092 antibody is able to block viral–host interactions. Only ~970 Å 2 of total molecular surface is buried in the F045–092–Vic1975/H3 interaction, divided evenly between HA and the Fab, and is the smallest footprint for any HA–antibody complex to date ( Supplementary Table 2 ). Figure 1: Antibody F045–092 binds the influenza HA receptor-binding site. Crystal structures of F045–092 Fab in complex with ( a ) Vic1975/H3 HA and ( b ) Vic2011/H3 HA. One Fab-HA protomer is coloured with HA1 in light blue, HA2 in green, the Fab heavy chain in purple and the Fab light chain in pink. Glycans are shown as spheres with carbon in yellow, oxygen in red and nitrogen in blue. ( c ) F045–092 binds HA using only its heavy chain and inserts its HCDR3 into the HA receptor-binding site. The HCDR3 contains a disulphide bridge, which is shown in yellow sticks. Full size image Figure 2: Receptor-binding site recognition by F045–092 to Vic1975/H3 in comparison to the α2,6 sialoglycan receptor. ( a ) F045–092 inserts its HCDR3 into the HA receptor-binding site. The carboxylate side chain of F045–092 Asp100e overlaps with the ( b ) carboxylate moiety of the sialic acid of the α2,6 sialoglycan receptor (PDB 2YP4) and uses identical hydrogen-bonding interactions, which are shown as black dashed lines. An additional hydrogen bond between the main chains of F045–092 and HA is circled in red dashed lines. The Leu100d side chain of F045–092 overlaps with the acetamide moiety of sialic acid. Full size image The VH1-69 germline is well known for producing heterosubtypic HA antibodies, which use a hydrophobic HCDR2 loop to target the stem of group 1 HAs [21] , [26] . However, other VH1-69 germline-encoded antibodies have been shown to insert their HCDR2 into the receptor-binding site [14] . F045–092 is also a VH1-69 germline-encoded antibody but primarily uses its HCDR3, which comprises 58% of the total surface area contributed by the Fab. The hydrophobic residues at the tip of HCDR2 (somatic Phe53 and germline Phe54) that are the hallmark of the VH1-69 family surprisingly only make minimal contacts with the outer ridges of the 150 loop and the 190 helix of HA. Sequence analysis of the F045–092 epitope To delineate the F045–092 binding determinants, the sequence of the HA epitope was analysed. F045–092 contacts a minimal epitope in and around the conserved receptor-binding site ( Fig. 3a ). Although F045–092 does indeed contact absolutely conserved residues involved in receptor recognition, the antibody also contacts some variable residues outside the receptor-binding site ( Fig. 3b ). The F045–092 epitope on the HA is quite variable across all human H3 strains and, at first glance, broad-spectrum recognition to a site with this relatively poor sequence conservation, apart from a handful of key residues that bind sialic acid, would not have been predicted as compared with the near absolute conservation of the HA stem-targeted epitopes [21] , [22] , [26] , [29] , [30] , [31] , [32] ( Fig. 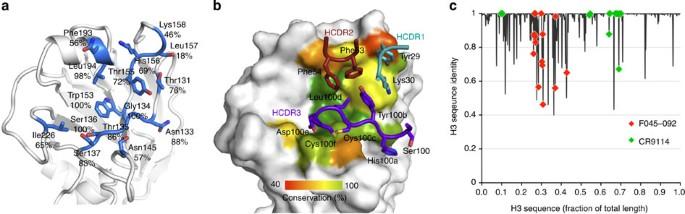Figure 3: Sequence conservation of the F045–092 epitope across human H3 viruses. (a) The F045–092 contact residues on HA are depicted as sticks. The per cent conservation for the most common residue found in the H3 subtype is labelled, which is not always identical to the residue at that position in the Vic1975/H3 sequence. (b) Interaction of F045–092 with Vic1975/H3 illustrating the sequence conservation of neutralizing epitope on the HA surface. For identification of the HA residues and positions that are colour coded on the surface, see (a). The F045–092 contact residues are labelled, coloured by HCDR, and shown as sticks. (c) Per cent identity of the most common residue among human H3 isolates plotted against the linear sequence of HA. Residues contacted by F045–092 or CR9114 are indicated by red or green diamonds, respectively. Although F045–092 contacts more hypervariable residues than CR9114 (but in different regions- head versus stem), it can still broadly neutralize the H3 subtype. 3c and Supplementary Table 3 ). Yet, F045–092 can tolerate natural variation in H3 strains that span from 1963 to 2011 ( Table 1 ). Furthermore, the current 2013–2014 H3 vaccine strain (A/Texas/50/2012) is antigenically similar to Vic2011/H3 and has an identical F045–092 epitope. Figure 3: Sequence conservation of the F045–092 epitope across human H3 viruses. ( a ) The F045–092 contact residues on HA are depicted as sticks. The per cent conservation for the most common residue found in the H3 subtype is labelled, which is not always identical to the residue at that position in the Vic1975/H3 sequence. ( b ) Interaction of F045–092 with Vic1975/H3 illustrating the sequence conservation of neutralizing epitope on the HA surface. For identification of the HA residues and positions that are colour coded on the surface, see ( a ). The F045–092 contact residues are labelled, coloured by HCDR, and shown as sticks. ( c ) Per cent identity of the most common residue among human H3 isolates plotted against the linear sequence of HA. Residues contacted by F045–092 or CR9114 are indicated by red or green diamonds, respectively. Although F045–092 contacts more hypervariable residues than CR9114 (but in different regions- head versus stem), it can still broadly neutralize the H3 subtype. Full size image Among the four loops that form the receptor-binding pocket, only the 150 loop does not contact the sialoglycan receptor and, therefore, it can accommodate high sequence variability as it is not functionally constrained for receptor recognition. Notwithstanding, the 150 loop contributes 40% of the total HA buried surface area in the F045–092–HA complex. However, the antibody appears to make non-specific interactions with the side chains of variable residues of HA such as with residues 156 and 158 that have a sequence conservation of 69% and 46% across all human H3 viruses, respectively ( Supplementary Fig. 3 ). Interactions with these and other variable residues appear to be permissive and do not create destabilizing clashes with F045–092, as the antibody is able to tolerate natural variation across decades of antigenic drift ( Table 1 ). In addition to the sequence variability in and around the receptor-binding site, insertions and deletions at or near the receptor-binding site loops can alter the conformations of the loops to evade immune recognition. In particular, the conformation of the 130 loop is important for F045–092 recognition as the antibody contacts this loop primarily through main-chain interactions and, thus, is not restricted by the natural variation of the residues in this loop in the H3 subtype. For instance, the 133a insertion (between residues 133 and 134) observed in ~78% of human H1 strains (observed in the 1918 and 2009 pandemic viruses) and in ~78% of human H5 strains produces a bulge in the 130 loop that protrudes from the receptor-binding site and would clash with F045–092 and other antibodies [12] , [16] , [17] . Notably, the H1 and H2 isolates recognized by F045–092 do not contain the 133a insertion. Also, a conserved two amino-acid insertion is present in the 150 loop of all H7 strains that likely will sterically prevent F045–092 binding. Although these idiosyncratic structural features of the receptor-binding loops limit the recognition of these particular strains and subtypes by F045–092 ( Supplementary Table 1 ), no insertions or deletions exist for any H3 strains, suggesting that sequence variation alone dictates immune evasion in the H3 subtype. HA glycan evasion In addition to continual antigenic drift, influenza HA can evade immune detection by masking neutralizing sites with glycans [33] , [34] , [35] , [36] , [37] . Within the H3 subtype, five conserved glycans exist at HA positions 22, 38, 165 and 285 on the HA1 subunit as well as 154 on HA2. Over time, H3 strains have incorporated and generally have retained several additional, potential N-linked glycosylation sites (PNGs) on the HA head ( Fig. 4a ). For example, Vic1975/H3 has seven PNGs per HA protomer, whereas Vic2011/H3 has these same seven and five additional PNGs in the HA head. This finding suggests that addition of glycans to H3 HAs is accretive, similar to the continual selection of variants in the HA amino-acid sequence by antigenic drift [38] . The added PNGs do not appear to occlude receptor binding but decorate the regions surrounding the receptor-binding site. Nevertheless, F045–092 evades these glycans to contact the HA protein surface. Most notably, a PNG in the 130 loop at Asn133 appeared in H3 viruses in 1996 and has been retained in successive viruses. As seen in the Vic2011/H3 complex, the glycan at this site is directed away from the receptor-binding site and does not interfere with F045–092 binding as the antibody slides in between the glycan and the HA 140 loop ( Fig. 4b ). Accordingly, the A/Panama/2007/1999 (H3N2) and A/Moscow/10/1999 (H3N2) strains, which have a PNG at Asn133, are both bound with very high affinity by the F045–092 Fab ( K d <20 nM). In addition, a PNG at Asn144 began to emerge in 1996, but no corresponding density for carbohydrate was observed in the Vic2011/H3 complex; however, the Asn side chain is directed away from the combining site ( Fig. 4b ) and suggests that potential glycosylation at this site would not obstruct F045–092 recognition, which is substantiated by the binding data. 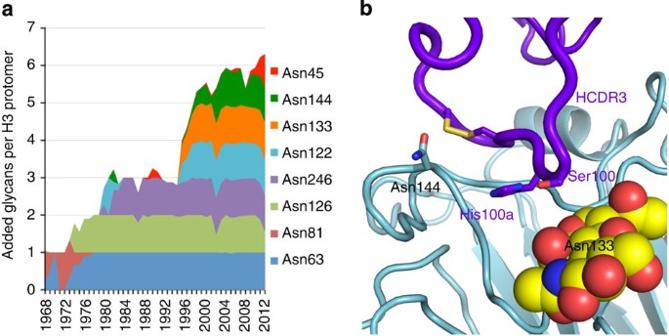Figure 4: Emergence of predicted N-linked glycans (PNGs) across human H3 viruses and evasion by F045–092. (a) Stacked graph showing the normalized percentage of strains that contain an additional PNG on HA1 at each indicated position. Seven PNGs have been incorporated in the HA since 1968 in addition to the five absolutely conserved PNGs in H3 strains (HA1 Asn22, Asn38, Asn165, Asn285; HA2 Asn154), except for the PNG at Asn81 (1968–1977). (b) F045–092 evades the glycan at Asn133 proximal to the receptor-binding site in the Vic2011/H3 complex. The glycan is shown as spheres, with carbon in yellow, oxygen in red and nitrogen in blue. No density corresponding to the PNG at Asn144 (shown as sticks) was observed. Figure 4: Emergence of predicted N-linked glycans (PNGs) across human H3 viruses and evasion by F045–092. ( a ) Stacked graph showing the normalized percentage of strains that contain an additional PNG on HA1 at each indicated position. Seven PNGs have been incorporated in the HA since 1968 in addition to the five absolutely conserved PNGs in H3 strains (HA1 Asn22, Asn38, Asn165, Asn285; HA2 Asn154), except for the PNG at Asn81 (1968–1977). ( b ) F045–092 evades the glycan at Asn133 proximal to the receptor-binding site in the Vic2011/H3 complex. The glycan is shown as spheres, with carbon in yellow, oxygen in red and nitrogen in blue. No density corresponding to the PNG at Asn144 (shown as sticks) was observed. Full size image F045–092 receptor mimicry The F045–092 HCDR3 adopts a protruding, blunt-ended conformation, which inserts into the receptor-binding site. The inserted residues include a disulphide loop consisting of residues Cys100c, Leu100d, Asp100e and Cys100f, which form a type I-like β turn. Remarkably, the side chains of the two central residues of the disulphide loop overlap with and chemically resemble sialic acid of the sialoglycan receptor ( Fig. 2 ). In particular, the isobutyl side chain of Leu100d aligns with the acetamide of sialic acid and similarly enters the hydrophobic pocket formed by the nearly universally conserved HA residues Trp153 and Leu194. Moreover, the carboxylate side chain of Asp100e closely aligns with the carboxylate of sialic acid and uses the same network of hydrogen bonds, including Ser136, which was predicted to contribute to antibody recognition [19] . Furthermore, the F045–092 HCDR3 curls over the 130 loop and creates an additional hydrogen bond between the Fab main chain at Tyr100b and HA1 Gly135 ( Fig. 2 ). The importance of the HCDR3 disulphide loop was investigated by alanine scanning mutagenesis. Individually mutating either Leu100d or Asp100e to alanine or eliminating the disulphide loop abolishes binding by F045–092 Fab to nearly every H3 strain tested ( Supplementary Table 4 ). These results suggest the identities of these four residues are the key determinants for F045–092 recognition of the H3 HA. Alanine mutagenesis of His100a, which is positioned in the groove between the 130 and 140 loops, does not have any major effect on the affinity of F045–092 to HA ( Supplementary Table 4 ). Its side chain is directed away from the HA and evades the glycan at Asn133 in the Vic2011/H3 complex ( Fig. 4b ). The residues that form and surround the vicinity of this groove, which is adjacent to the receptor-binding pocket, are highly conserved among H3 isolates ( Supplementary Fig. 4 ). This cleft may then be a potential secondary hotspot for the expansion of receptor-binding site directed small molecules or engineered proteins. Influenza H3N2 viruses have circulated in humans ever since the 1968 Hong Kong pandemic. In the span of nearly five decades, the H3 HAs have diverged by antigenic drift so that the current H3 strain has only ~80% sequence identity to the 1968 H3 strain, with the majority of that variation focused in the HA head. In addition, glycans are periodically incorporated and retained as an immune evasion strategy employed by H3 viruses to shield antigenic sites [33] , [34] . The extent of the additional masking of the HA surface by glycans from 1968 to present can be clearly visualized in the Vic2011/H3 HA structure ( Supplementary Fig. 5 ). The crystal structures of heterosubtypic, pan-H3 antibody F045–092 in complex with the HAs from 1975 and 2011 H3N2 viruses reveal how the antibody can broadly neutralize the H3 subtype through insertion of a long HCDR3 loop into the HA receptor-binding site. Although F045–092 does not make specific contacts with the HA glycans around the receptor-binding site but rather avoids them, its mode of binding to HA resembles to some extent the exceptionally long HCDR3 loops of many anti-HIV antibodies, especially those that use their HCDR3 loops to reach into recessed sites or penetrate through the glycan shield of HIV-1 Env to contact the protein surface below [39] , [40] , [41] , [42] . The principal contacts of F045–092 to the HA are via HCDR3, which contains a disulphide loop. The antibody binds a minimal HA epitope that is located in and around the receptor-binding site and has the smallest footprint on HA to date ( Supplementary Table 2 ). The HCDR3 Asp100e and Leu100d, which are between the Cys residues (Cys100c, Cys100f) that form the disulphide loop, mimic the hydrogen-bonding network of the carboxylate and the hydrophobic acetamide moiety of the endogenous sialoglycan receptor, respectively, and are critical for antibody recognition to the HA. Furthermore, an additional hydrogen bond is formed between the main chains of F045–092 and the HA 130 loop, which represent an interaction that sialoglycan receptors do not utilize. Yet, due to the larger footprint of the antibody on HA (~490 Å 2 ) compared with sialic acid (~190 Å 2 ), it is inevitable that F045–092 will contact some non-conserved residues outside the receptor-binding site. However, F045–092 is able to overcome the antigenic variation of the H3 subtype, as well as the addition and accumulation of glycans, surrounding the receptor-binding site and binds some HA strains with a K d ~nM as compared with a K d ~mM for the sialoglycan receptor, a difference of six orders of magnitude. Studies [43] indicate that H3 strains with increased glycosylation have significantly decreased affinity for receptor, particularly in strains that appeared around and after 2003 and, in accord, the F045–092 Fab exhibits weaker binding for these more recent H3 strains ( Table 1 ). However, the antibody binding appears to be tuned such that weaker Fab binding can be enhanced and accommodated by avidity of the bivalent IgG so as to extend the antibody’s breadth of recognition, as observed with some other receptor-binding-site-targeted antibodies [15] , [16] , [17] . In addition, F045–092 appears to use slightly different approach angles to bind the Vic1975/H3 and Vic2011/H3 HAs, pivoting around the receptor-binding site likely to accommodate variable epitope residues. Altogether, these binding features allow F045–092 to have exceptional binding breadth against the entire H3 subtype as well as strains from the H1, H2 and H13 subtypes. Common trends of recognition, as seen with F045–092 and other antibodies, are now emerging that show recurring modes of binding to attain broad recognition of the receptor-binding site. For instance, the use of receptor mimicry has been observed in other antibodies that similarly insert their HCDR3 into the HA receptor-binding site, which all use an Asp carboxylate at the tip of the loop to mimic the carboxylate of sialic acid [12] , [13] , [15] , [44] , [45] . These findings suggest that receptor mimicry of the carboxylate may be important for broad recognition of HA, which is utilized by half of the receptor-binding-site-targeted antibodies solved in complex with HAs to date ( Fig. 5a ), although other antibodies recognize this portion of the receptor-binding site by other means [14] , [16] , [17] , [23] . In addition, nearly all receptor-binding-site-targeted antibodies commonly insert a hydrophobic residue into the universally conserved hydrophobic pocket formed by Trp153 and Leu194 that would be occupied by the acetamide moiety of sialic acid. The identity of this hydrophobic residue can vary from a smaller residue, such as proline or valine, to a bulky aromatic residue, such as tyrosine, phenylalanine or tryptophan ( Fig. 5b ). Among the structurally characterized receptor-binding-site-targeted antibodies, F045–092 most closely resembles C05 as both antibodies contact a very small HA footprint primarily through their long HCDR3 loops [16] . In contrast, these antibodies differ in their angle of approach by ~113° ( Supplementary Fig. 6 ) and the interaction of C05 with HA does not resemble those of the receptor, suggesting that there is considerable versatility in targeting the receptor-binding site. 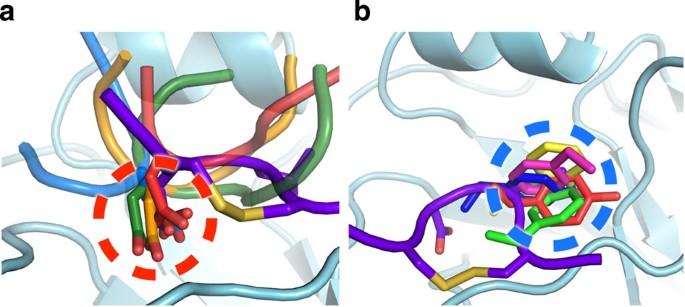Figure 5: Common trends in recognition of the HA by receptor-binding-site-targeted antibodies. (a) Antibodies HC19 (red, PDB 2VIR), HC63 (light blue, PDB 1KEN), CH65 (green, PDB 3SM5) and 5J8 (orange, PDB 4M5Z) use an Asp residue to insert a carboxylate in the receptor-binding site that would be occupied by the carboxylate of sialic acid of the α2,6 sialoglycan receptor (dashed red circle). (b) Antibodies HC19 (red, PDB 2VIR), C05 (yellow, PDB 4FP8), 8F8 (blue, PDB 4HF5), 8M2 (pink, PDB 4HFU) and 2G1 (green, PDB 4HG4) use hydrophobic residues to target the receptor-binding site that would be occupied by the acetamide moiety of sialic acid (dashed blue circle). The disulphide loop of the F045–092 HCDR3 is shown and coloured purple. Figure 5: Common trends in recognition of the HA by receptor-binding-site-targeted antibodies. ( a ) Antibodies HC19 (red, PDB 2VIR), HC63 (light blue, PDB 1KEN), CH65 (green, PDB 3SM5) and 5J8 (orange, PDB 4M5Z) use an Asp residue to insert a carboxylate in the receptor-binding site that would be occupied by the carboxylate of sialic acid of the α2,6 sialoglycan receptor (dashed red circle). ( b ) Antibodies HC19 (red, PDB 2VIR), C05 (yellow, PDB 4FP8), 8F8 (blue, PDB 4HF5), 8M2 (pink, PDB 4HFU) and 2G1 (green, PDB 4HG4) use hydrophobic residues to target the receptor-binding site that would be occupied by the acetamide moiety of sialic acid (dashed blue circle). The disulphide loop of the F045–092 HCDR3 is shown and coloured purple. Full size image The crystal structures of F045–092 in complex with divergent HAs reveal that the receptor-binding site is a hotspot for antibody recognition and is a key site of vulnerability against influenza HA. The challenge now is how the information gained from these structures can be applied to inform the design of improved vaccines or broad-spectrum small-molecule therapeutics, which are currently unavailable as a countermeasure against influenza HA. For instance, multimerization of the HA heads onto a self-assembling platform in combination with epitope focusing of the receptor-binding site may elicit a greater antibody response as an alternative vaccination strategy [46] , [47] . Since F045–092 only uses its V H domain to contact a very minimal epitope on HA, it may be a promising candidate as a nanobody therapeutic or a diagnostic against H3 viruses [48] , [49] . Owing to its extremely small footprint on HA, another possibility may be to computationally design small proteins to bind the receptor-binding site, as previously achieved for the HA stem [50] , [51] . However, the synthesized F045–092 HCDR3 peptide does not compete with Fab binding nor could it be co-crystallized with HA, suggesting that the antibody stabilizes the proper conformation of the antibody HCDR3 loop by utilizing contacts from the other HCDRs, as also seen for the C05 antibody [16] . Although the ultimate goal is for universal therapy against all flu viruses, it may be more practical to also focus attention on the H1, H3 and flu B viruses that currently circulate in humans and have been responsible for all recent pandemics, epidemics and seasonal flu in the last 46 years. No previous antibody has been able to achieve complete HA subtype recognition at the receptor-binding site as described and characterized here for F045–092, and the structural information has great potential to serve as a template for the design of next-generation therapeutics against all H3 influenza viruses. Fab and IgG expression and purification F045–092 Fab and Fab mutants (His H100a Ala; Cys H100c Ala, Cys H100f Ala; Leu H100d Ala; Asp H100e Ala) were individually cloned into the pFastBac Dual vector (Invitrogen) with N-terminal gp67 signal peptides fused to the light and heavy chains and a C-terminal His 6 tag fused to the heavy chain. Recombinant bacmid DNA was generated using the Bac-to-Bac system (Invitrogen) and baculovirus was generated by transfecting purified bacmid DNA into Sf9 cells using Cellfectin II (Invitrogen). F045–092 Fab and mutants were expressed by infecting suspension cultures of High Five cells (Invitrogen) with baculovirus shaking at 110 r.p.m. for 72 h at 28 °C. The proteins were purified by Ni-NTA (Qiagen), protein G, Mono S chromatography (GE Healthcare), followed by a final step of gel filtration (GE Healthcare). F045–092 Fab was also prepared in E. coli DH12S cells (Invitrogen). C-terminal His 6 and FLAG tags were fused to the heavy and light chains, respectively. DH12S cells harbouring the F045–092 Fab expression plasmids were cultured in 2 × YT medium at 30 °C and induced with 1 mM IPTG at an optical density of 0.7 overnight. The culture supernatant was recovered and subjected to 60% ammonium sulphate precipitation. The precipitant was dissolved in PBS and the Fab was purified by Ni-NTA (Qiagen), anti-FLAG antibody M2 (Sigma), Mono S chromatography (GE Healthcare), followed by a final step of gel filtration (GE Healthcare). To generate F045–092 IgG, the antibody light and heavy chains were each cloned into a modified pCAGGS vector [52] containing a dihydrofolate reductase (DHFR) gene. CHO (DHFR−) cells were co-transfected with the resultant plasmids and cultured in serum-free media. F045–092 IgG was purified from the culture supernatant by Capto Q chromatography (GE Healthcare) and Protein A affinity chromatography (ProteNova). HA expression and purification Baculovirus-expressed HA was prepared for binding studies and crystallization. Briefly, each HA was fused with an N-terminal gp67 signal peptide and a C-terminal BirA biotinylation site, thrombin cleavage site, trimerization domain and a His 6 tag. The HAs were expressed, as described above for the F045–092 Fabs, as either HA0 (human HAs) or mature HA (HA1/HA2; due to the polybasic linker in avian HAs between HA1 and HA2) and purified by Ni-NTA (Qiagen). For crystallization, the HA0 of Vic1975/H3 was treated with trypsin (NEB) to remove the C-terminal foldon and His 6 tags and to produce mature HA. The HA was then purified by a final step of gel filtration (GE Healthcare). For binding studies, each HA0 or mature HA was biotinylated with BirA and purified by gel filtration (GE Healthcare). The biotinylation reactions contained 100 mM Tris (pH 8.0), 10 mM ATP, 10 mM magnesium acetate, 50 μM biotin and <50 mM NaCl, and were incubated at 37 °C for 1–2 h. K d determination K d values were determined by bio-layer interferometry using an Octet RED instrument (ForteBio, Inc.). Biotinylated HAs at ~10–50 μg ml −1 in 1 × kinetics buffer (1 × PBS (pH 7.4), 0.01% BSA and 0.002% Tween 20) were immobilized onto streptavidin-coated biosensors and incubated with varying concentrations of baculovirus-expressed F045–092 Fab or IgG. All binding data were collected at 30 °C. The k on and k off values of each Fab and IgG were measured in real-time to determine K d values for each Fab and IgG for each HA tested. The sequences of the HA proteins used in the binding studies and the experimental binding curves for each Fab and IgG for fitting k on and k off are reported in Supplementary Fig. 7 . The sequences of all biotinylated HAs used in this work are available in FASTA format in the Supplementary Methods . Crystallization and structural determination of Fab F045–092 Bacterially expressed F045–092 Fab crystals were grown by sitting-drop vapour diffusion at 20 °C by mixing 0.75 μl of concentrated protein sample (7.3 mg ml −1 ) with 0.75 μl of mother liquor (30% PEG 600, 0.1 M phosphate-citrate, pH 5.0). Crystals appeared in 7 days and were cryoprotected with mother liquor supplemented with 20% ethylene glycol. X-ray diffraction data were collected to 1.50 Å resolution at beamline 11-1 (wavelength 0.97945 Å) at the Stanford Synchrotron Radiation Lightsource (SSRL) and were processed in space group P2 1 2 1 2 1 using XDS [53] . The structure was determined by molecular replacement with Phaser [54] using the variable and constant domains of Fab New (PDB 7FAB (ref. 55 )) as search models and one Fab was found in the asymmetric unit. The model was iteratively rebuilt using Coot [56] and refined in Phenix [57] . Refinement parameters include initial rigid-body refinement (each Ig domain) and simulated annealing followed by restrained refinement including TLS refinement (each Ig domain as a TLS group). In the final F045–092 Fab structure, 97.9% of the residues are in favored regions of the Ramachandran plot with 0% outliers, as calculated by MolProbity [58] . Crystallization and structural determination of the Vic2011/H3 HA EndoH-treated baculovirus-expressed Vic2011/H3 HA was crystallized by sitting-drop vapour diffusion at 4 °C by mixing 0.75 μl of concentrated protein sample (3 mg ml −1 ) with 0.75 μl of mother liquor (5% PEG 8000, 20% PEG 300, 10% glycerol, 0.1 M Tris, pH 8.7). Crystals appeared in 3 days. X-ray diffraction data were collected to 1.75 Å resolution at SSRL beamline 11-1 (wavelength 0.97945 Å) and were processed in space group H32 using XDS [53] . The structure was determined by molecular replacement with Phaser [54] using a protomer of the apo 2005 Hong Kong (H3N2) HA (PDB 2YP7 (ref. 43 )) as the search model. One HA protomer (HA1/HA2) of the HA trimer was found in the asymmetric unit. The model was iteratively rebuilt using Coot [56] and refined in Phenix [57] . Refinement parameters include initial rigid-body refinement and simulated annealing followed by restrained refinement including TLS refinement (each HA1 and HA2 chain). In the final Vic2011/H3 HA structure, 96.6% of the residues are in favored regions of the Ramachandran plot with 0% outliers [58] . Crystallization and structural determination of F045–092 Fab-HA complexes For Fab–HA complex formation, baculovirus-expressed Fab F045–092 was added to Vic1975/H3 or Vic2011/H3 HA in a molar ratio of 3.2:1 to achieve 3 Fabs per HA trimer, incubated at room temperature for 1 h and the complex was then purified from unbound Fab by gel filtration. F045–092–Vic1975/H3 crystals were grown by sitting drop vapour diffusion at 4 °C by mixing 0.75 μl of concentrated protein sample (5.7 mg ml −1 ) with 0.75 μl of mother liquor (1.7 M ammonium sulphate, 0.1 M Tris (pH 8.1), 4% PEG 400). Crystals appeared in 7 days and were cryoprotected with mother liquor supplemented with increasing concentrations of glycerol (5% steps, 10 min per step) to a final concentration of 25%. X-ray diffraction data were collected to 2.75 Å resolution at the GM/CA CAT 23ID-B beamline (wavelength 1.03322 Å) at the Advanced Photon Source (APS) and were processed in space group P321 using XDS [53] . The structure was determined by molecular replacement with Phaser [54] , using the variable domain of the high-resolution Fab structure and the HA protomer of Vic1975/H3 (PDB 4GMS (ref. 17 ), chains A and B) as models. After rigid-body refinement of the HA and Fab variable domain, density was observed for the constant domain, which was docked in by hand and refined using rigid-body refinement. The model was iteratively rebuilt using Coot [56] and refined in Phenix [57] . Refinement parameters include rigid-body refinement (each Ig domain and HA protomer) and simulated annealing followed by restrained refinement including TLS refinement (each Ig domain and HA chain). In the final F045–092–Vic1975/H3 structure, 96.2% of the residues are in favored regions of the Ramachandran plot with 0.3% outliers [58] . F045–092–Vic2011/H3 crystals were grown by sitting-drop vapour diffusion at 20 °C by mixing 0.75 μl of concentrated protein sample (9.1 mg ml −1 ) with 0.75 μl of mother liquor (20% PEG 400, 30% 1,2-propanediol, 0.1 M HEPES, pH 7.5). Crystals appeared in 7 days. X-ray diffraction data were collected to 6.50 Å resolution at the GM/CA CAT 23ID-B beamline (wavelength 1.03318 Å) at APS and were processed in space group C2 using XDS [53] . The structure was determined by molecular replacement with Phaser [54] using the high-resolution apo A/Victoria/361/2011 (H3N2) HA trimer as a search model to locate two HA trimers in the asymmetric unit. Next, six copies of the variable domain of the high-resolution F045–092 Fab structure were used as search models after fixing the position and orientation of the two HA trimers but only five variable domain copies were found. After rigid-body refinement, density was observed for the remaining Fab variable and constant domains, which were then docked in by hand and refined with rigid-body refinement. The model was iteratively rebuilt using Coot [56] and refined in Phenix [57] using the high-resolution Fab and HA structures to generate reference model restraints and with similar parameters as in the F045–092–Vic1975/H3 complex. In the final F045–092–Vic2011/H3 structure, 97.4% of the residues are in favored regions of the Ramachandran plot with 0% outliers [58] . The data were processed and the structure was refined in a C2 space group but exhibited pseudosymmetry that resembled the symmetry in space group P321. However, the C2 space group appeared to be the correct choice and also had better statistics and better density, especially for some of the carbohydrate moieties. Structural analyses Hydrogen bonds and van der Waals contacts were calculated using HBPLUS [59] and CONTACSYM [60] , respectively. Molecular surface area buried upon Fab binding was calculated using MS [61] . MacPyMol (DeLano Scientific) was used to render structure figures. Kabat numbering was applied to the variable domains of the Fabs using the AbNum server [62] . The final coordinates were validated using the JCSG quality control server (v2.8), which includes MolProbity [58] . Sequence analysis of F045–092 epitope conservation All full-length and non-redundant human influenza A HA sequences were downloaded on 12 December 2013 from the Influenza Virus Resource at the NCBI database [63] . The sequences were aligned using MUSCLE [64] and analysed using GCG (Accelrys) and custom shell scripts (available from the authors upon request). Accession codes: Coordinates and structure factors have been deposited in the RCSB Protein Data Bank under accession codes 4O58 (F045–092–Vic1975/H3 complex), 4O5I (F045–092–Vic2011/H3 complex), 4O5L (apo F045–092 Fab) and 4O5N (apo Vic2011/H3 HA). How to cite this article: Lee, P. S. et al. Receptor mimicry by antibody F045–092 facilitates universal binding to the H3 subtype of influenza virus. Nat. Commun. 5:3614 doi: 10.1038/ncomms4614 (2014).